Shared rules of development predict patterns of evolution in vertebrate segmentation Phenotypic diversity is not uniformly distributed, but how biased patterns of evolutionary variation are generated and whether common developmental mechanisms are responsible remains debatable. High-level ‘rules’ of self-organization and assembly are increasingly used to model organismal development, even when the underlying cellular or molecular players are unknown. One such rule, the inhibitory cascade, predicts that proportions of segmental series derive from the relative strengths of activating and inhibitory interactions acting on both local and global scales. Here we show that this developmental design rule explains population-level variation in segment proportions, their response to artificial selection and experimental blockade of putative signals and macroevolutionary diversity in limbs, digits and somites. Together with evidence from teeth, these results indicate that segmentation across independent developmental modules shares a common regulatory ‘logic’, which has a predictable impact on both their short and long-term evolvability. A major goal of evolutionary developmental biology is to identify whether there are rules governing the generation of phenotypic variation and how these might impact evolvability [1] . Some of the most recognizable evolved differences among taxa are variations in the number and/or size of iterative segments such as teeth [2] , limbs [3] , phalanges [4] and somites [5] . Despite apparent diversity, evidence suggests that developmental interactions create predictable, non-random patterns of variation (for example, in digits [4] and limbs [6] ). While morphogenesis of each of these organ systems utilizes similar developmental processes of ‘outgrowth and segmentation’ [7] , [8] , [9] , a lack of genetic and structural homology among them has led to the presumption that different developmental principles must apply to each system. Commonalities in regulatory ‘logic’ may predict similar underlying ‘rules’ of variation even when the underlying identity of cellular or molecular players differs [10] , [11] , [12] , [13] . One such model, the inhibitory cascade (IC) [14] , is particularly promising for understanding iterative segmentation in a range of disparate organ systems. Originally described in teeth, the IC can be generalized to any sequentially forming structure that develops at the balance between auto-regulatory ‘activator’ and ‘inhibitor’ signals. In, limbs [15] and somites [16] , such signals are analogous to internal ‘clock’-like mechanisms posited to control timing of condensation formation and molecular gradients or ‘wavefronts’ that inhibit them. In contrast to previous models, the IC makes explicit quantitative predictions of how proportional variation is apportioned among segments, thus both comparative and experimental data from segmented structures can be used as direct tests. Specifically, the IC can be modelled by equation (1): Where s is a segment, n is the segment position expressed as an integer, a is the activator strength and i is the inhibitor strength [15] . Assuming a linear effect of activator to inhibitor, solving equation (1) for a three-segment system yields sizes of: [ s 1 ]=1, and . Expressed as proportions, equation (1) further predicts that for a three-segment system the middle segment is one-third the total size (that is, , , and (see Methods)), the proximal and distal segment proportions function as a tradeoff that accounts for the remainder (that is, s n +2 =−1·s n +2/3) and the ratio of the size of the first two segments predicts the ratio of the first and third (that is, [ s n +2 / s n ]=2·[ s n +1 / s n ]−1). 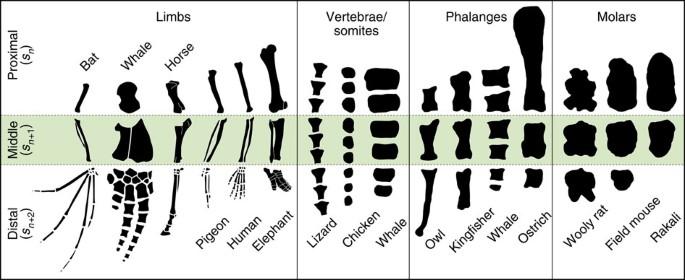Figure 1: Iteratively segmented structures exhibit similar variational features predicted by the inhibitory cascade model. The middle segment averages one-third of total size and exhibits reduced variance, while proximal and distal segment proportions function as a tradeoff for any series of three adjacent individual segments or blocks of segments. From left to right, example specimens include: a bat wing (Carollia perspicillata), dolphin flipper (Tursiops truncatus), horse forelimb (Equus ferus caballus), pigeon wing (Columbia livia), human arm (Homo sapiens), elephant hindlimb (Loxodonta africana), lizard vertebrae (Varanus indicus), chick somites (Gallus gallus), humpback whale tail vertebrae (Megaptera novaeangliae), Saw whet owl foot digit III phalanges (Aegolius acadicus), Kingfisher foot digit III phalanges (Alcedo atthis), Whale forelimb phalanges (Megaptera novaeangliae), ostrich foot digit III phalanges (Struthio camelus) Woolly rat molars (Mallomys rothschildi), field mouse molars (Apodomus agrarius) and Rakali rodent molars (Hydromys chrysogaster). The IC model can be further extended to predict sizes and proportions for any total number of segments (see Supplementary Table 1 ). Importantly, equation (1) can be generalized such that any three adjacent segments or blocks of segments (the ‘local’ effect) within a series are predicted to exhibit the same behaviour regardless of the total segment number (see Methods). Because the overall pattern (the ‘global effect) results from the sum of local effects from all adjacencies, the partitioning of total variance is reflected in a parabolic relationship with total segment number, with the middle segment(s) at the vertex or minima and equivalent to either 1/ n (when odd numbered) or 2/ n (when even numbered). As with the three-segment solution, the proximal-most and distal-most segments or blocks receive the most variance, and proportions act as a ‘tradeoff’, which is further reflected in diagnostic covariation among individual segment proportions. If the IC is a generalizable developmental rule, then it should be able to predict how size proportion variation is both structured within populations and responds to selection or experimental perturbations in a range of segmented structures. Furthermore, because biases in the generation of variation impact evolvability [17] , the signal of this mechanism would be evident in the patterning of macroevolutionary diversity among species ( Fig. 1 ). As alternative ‘rules’ for generating proportions, we modelled segment variation in which the strength of size covariation ranged from 0 (that is, completely random) to 1 in which segment sizes had a constant directionality (that is, they did not alternate), but the amount is random between segments. These alternatives predicted outcomes distinct from the IC, such as: (1) all types of segment proportions occur with equal frequency, (2) normalized variances are non-parabolic and (3) relationships between adjacent segments are weaker and more distributed. In this context, the IC model represents a specific subset of these alternatives, in which activator–inhibitor interactions are constant among segments. Figure 1: Iteratively segmented structures exhibit similar variational features predicted by the inhibitory cascade model. The middle segment averages one-third of total size and exhibits reduced variance, while proximal and distal segment proportions function as a tradeoff for any series of three adjacent individual segments or blocks of segments. From left to right, example specimens include: a bat wing ( Carollia perspicillata ), dolphin flipper ( Tursiops truncatus ), horse forelimb ( Equus ferus caballus ), pigeon wing ( Columbia livia ), human arm ( Homo sapiens ), elephant hindlimb ( Loxodonta africana ), lizard vertebrae ( Varanus indicus ), chick somites ( Gallus gallus ), humpback whale tail vertebrae ( Megaptera novaeangliae ), Saw whet owl foot digit III phalanges ( Aegolius acadicus ), Kingfisher foot digit III phalanges ( Alcedo atthis ), Whale forelimb phalanges ( Megaptera novaeangliae ), ostrich foot digit III phalanges ( Struthio camelus ) Woolly rat molars ( Mallomys rothschildi ), field mouse molars ( Apodomus agrarius ) and Rakali rodent molars ( Hydromys chrysogaster ). Full size image Here we test the quantitative predictions of the IC model in developmental experiments, species under artificial selection, and microevolutionary and macroevolutionary data sets of segmented structures including limbs, phalanges, somites and vertebrae. We find that all these systems follow the expectations of the model, including predictable variation of size proportions, a proximo-distal trade-off in size and variance apportioned parabolically. These widely shared segmentation rules raise questions about the extent of developmental bias in the structural design of animal bodies. The IC model predicts experimental outcomes in phalanges We first tested model predictions in digits by quantifying phalangeal proportions in normal chicken ( Gallus gallus ) embryos immediately post-patterning ( Supplementary Data 1 ). We found they followed the expectations of the IC model, with a proximo-distal tradeoff ( s n +2 =−1.00 × s n +0.70, r 2 =0.790, P <0.001), significantly lower variation in the middle segment (Levene’s test, P <0.001) and a mean just under ~1/3 of proportions ( s n +1 =0.297±0.023) ( Fig. 2a ). Next, we tested the IC model prediction that altering the relative balance of the strength of activation to inhibition would affect segmental outcomes and proportions. We reasoned that, even without a priori knowledge of the exact signals involved, if segments were generated via an activator–inhibitor dynamic interaction, an impermeable barrier would alter their balance and phenotypic outcomes. Specifically, we hypothesized that if s 1 plays an inhibitory role on subsequent s 2 , then by disrupting the signal between them we would see a shift in proximo-distal proportions of the downstream s 2 – s 3 – s 4 series. Consistent with these predictions, we observed that even when controlled for reductions in total size (sum of all phalanges within a digit), the barrier significantly increased proximal s 2 proportions relative to controls (from 0.422±0.024 to 0.448±0.048, analysis of covariance (ANCOVA), P <0.001) and decreased distal s 4 proportions (from 0.286±0.025 to 0.250±0.024, ANCOVA, P <0.001), but in all cases left the middle segment [ s 3 ] statistically unchanged (0.292±0.013 to 0.300±0.016, ANCOVA, P =0.433; Fig. 2b ). Moreover, experimental, control and wild-type segment proportions share a common proximo-distal trajectory (likelihood ratio=3.391, df=2, P =0.184) that is statistically indistinguishable from model prediction ( s n+2 =−0.97 × s n +0.69, r 2 =0.813, P <0.001; r =−0.063, df=199, P =0.375). 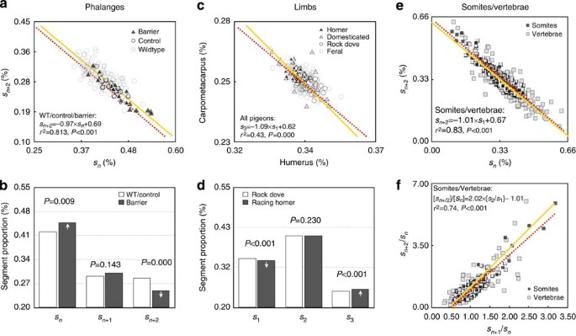Figure 2: Normal population-level and induced variation is consistent with predictions of an inhibitory cascade. (a) Proximal-distal tradeoffs in experimental groups are statistically indistinguishable from wildtype/controls (likelihood ratio=3.391, df=2,P=0.184), and together they are consistent with IC model predictions (yellow line:sn+2=−0.97 ×sn+0.69,r2=0.813,P=0.000;r=−0.063, df=199,P=0.375). (b) An impermeable barrier between developing thes0–snjoint leads to a significant increase in proximal phalangeal proportions (sn) and decrease in distal segment (sn+2) proportions, while middle segment (sn+1) proportions remain unchanged (ANCOVA,P<0.001). (c) The rock dove (Columba livia) and domesticated/feral pigeons follow the same proximal-distal tradeoff (yellow), paralleling the predicted IC model trajectory (red dashed) (r=0.060, df=34,P=0.729). (d) The ‘Racing Homer’ domesticated pigeon breed has significantly shifted proximal-distal (s1–s3) wing element proportions, but no difference was found in zeugopod (s2) proportion (ANCOVA,P<0.001,N=54). Note that digits were not included in this analysis, thuss2proportions are inflated, but otherwise does not impact thes1–s3tradeoff prediction. (e,f) When decomposed into local three-segment series, somites and their skeletal derivatives (principally vertebral centra) exhibit a PD trajectory consistent with the IC model predictions (sn+1=0.331±0.001;sn+2=−1.01 ×s1+0.67,r2=0.83,P<0.001; [sn+/2]/[sn] = 2.02 × [s2/s1]−1.01,r2=0.74,P<0.001). Figure 2: Normal population-level and induced variation is consistent with predictions of an inhibitory cascade. ( a ) Proximal-distal tradeoffs in experimental groups are statistically indistinguishable from wildtype/controls (likelihood ratio=3.391, df=2, P =0.184), and together they are consistent with IC model predictions (yellow line: s n+2 =−0.97 × s n +0.69, r 2 =0.813, P =0.000; r =−0.063, df=199, P =0.375). ( b ) An impermeable barrier between developing the s 0 – s n joint leads to a significant increase in proximal phalangeal proportions ( s n ) and decrease in distal segment ( s n +2 ) proportions, while middle segment ( s n +1 ) proportions remain unchanged (ANCOVA, P <0.001). ( c ) The rock dove ( Columba livia ) and domesticated/feral pigeons follow the same proximal-distal tradeoff (yellow), paralleling the predicted IC model trajectory (red dashed) ( r =0.060, df=34, P =0.729). ( d ) The ‘Racing Homer’ domesticated pigeon breed has significantly shifted proximal-distal ( s 1 – s 3 ) wing element proportions, but no difference was found in zeugopod ( s 2 ) proportion (ANCOVA, P <0.001, N =54). Note that digits were not included in this analysis, thus s 2 proportions are inflated, but otherwise does not impact the s 1 – s 3 tradeoff prediction. ( e , f ) When decomposed into local three-segment series, somites and their skeletal derivatives (principally vertebral centra) exhibit a PD trajectory consistent with the IC model predictions ( s n+1 =0.331±0.001; s n+2 =−1.01 × s 1 +0.67, r 2 =0.83, P <0.001; [ s n+/2 ]/[ s n ] = 2.02 × [ s 2 / s 1 ]−1.01, r 2 =0.74, P <0.001). Full size image The IC model predicts microevolution of limb segment size proportions We next analysed intraspecific variation in the forelimbs (wings) of the adult rock dove ( Columba livia ). Consistent with the IC model predictions, we found that rock dove proximal-distal wing proportions ( s 3 =−1.06 × s 1 +0.61, r 2 =0.184, P =0.009) are not significantly different from the predicted tradeoff slope ( r =0.060, df=34, P =0.729) or intercept ( t =−1.026, df=34, P =0.312; Fig. 2c ). We next compared these results to domesticated pigeon breeds and related ferals ( C. livia domestica ; Supplementary Data 2 ). Pigeons have been domesticated for at least 10,000 years, with breeders targeting a range of phenotypic traits, including overall body size and limb length, while ferals are domesticated pigeons that have escaped into the wild and populated novel ecological niches [18] and maintain significant gene flow introgression [19] . We reasoned that the effect of selection and population expansion would be to increase variation in these groups, but along a trajectory consistent with rock doves and the IC model. Indeed, when compared with rock doves, in both domesticated ( s 3 =−1.24 × s 1 +0.67, r 2 =0.45) and feral groups ( s 3 =−1.06 × s 1 +0.61, r 2 =0.38) there was no significant difference in slope (likelihood ratio=1.679, df=2, P =0.432) or elevation (Wald Statistic=1.304, df=2, P =0.520) although both groups were significantly shifted along this common axis (Wald Statistic=85.53, df=2, P =0.000). Relevant to this final observation, one breed in particular, the ‘Racing Homer’, has been selectively bred in the last 100 years for speed, and relative to the rock dove, is significantly shifted in proximal-distal proportions (humerus: 0.343±0.002 versus 0.337±0.002, ANCOVA, P <0.001; carpo-metacarpus: 0.254±0.002 versus 248±0.002, ANCOVA, P <0.001, N =54), yet the zeugopod is not significantly different in proportions, even when controlled for differences in wing length ( P =0.232) ( Fig. 2d ). These results indicate that selection on size alone cannot explain the observed changes in homer wing proportions; rather selective breeding has evolved proportions along a line of developmental ‘least resistance’ present within ancestral rock doves and predicted by the IC model. The IC model predicts variation of somites and their derivatives We next asked whether variation in somites is also consistent with quantitative predictions of the IC model using available data. Previous reports suggest somites form as an antero-posterior gradient in which sizes do not alternate (for example, increasing size in mice [20] , decreasing size in amphibians [21] or equal size in avians [22] ). Analysis of the somite data matches those of the IC predictions (s n +1 =0.325±0.001; s n +2 =−1.00·s n +0.67, r 2 =0.935, P <0.001; [ s n +2 ]/[ s n ]=2.10·[ s n +1 ]/[ s n ]−1.03, r 2 =0.932, P <0.001) ( Supplementary Data 3 ; Fig. 2e ). As a further test, we analysed vertebral column proportions in primates, rodents, carnivores and amphibians. Although individual vertebrae are derived from adjacent somites, we reasoned that if each vertebra forms from one half of two adjacent somites and if growth of adjacent vertebrae were similar, then the local pattern (that is, among any three adjacent segments or blocks) should follow the IC model. Indeed, we found that when decomposed into local adjacencies or blocks, combined data from the vertebral columns were consistent with the IC model tradeoff (s n +1 =0.332±0.001; s n +2 =−1.01·s n +0.67, r 2 =0.810, P <0.001; [ s n +2 ]/[ s n ]=1.98·[ s n +1 ]/[ s n ]−0.97, r 2 =0.651, P <0.001) Supplementary Data 3 ; Fig. 2f ). The IC model predicts macroevolutionary diversity An IC mechanism should also impact evolvability, which on a macroevolutionary scale would be reflected in biased distributions of species-level segment proportions along a common ‘line of least resistance’, in this case the proximal-distal tradeoff [14] , [23] . Limbs, phalanges and somites exhibit a range of proximo-distally arranged total segments, from 3 (for example, in limbs and most mammalian digits) to as many as 28 (for example, in the digits of ichthyosaurs or in vertebral columns) ( Supplementary Data 4–11 ). We first compared limb data, which have three defined segments, to digital rays that numbered three total phalangeal segments. We found that these data sets had similar properties to those predicted by the IC model, including a middle segment proportion centre of ~1/3 (digit: s 2 =0.334±0.037, limb: s 2 =0.356±0.014) with significantly reduced variance relative to proximal and distal segments (Levene’s test, P <0.001) ( Supplementary Tables 2a–c ). Furthermore, proximal and distal segment proportions operated as a tradeoff (limb: s 3 =−1.05·s 1 +0.67, r 2 =0.793, P =0.000; digit: s 3 =−0.93·s 1 +0.65, r 2 =0.671, P =0.000) ( Supplementary Fig. 4a–d ), with elevations statistically indistinguishable from the IC model (limb: t =−0.035, df=826, P =0.972; digit: t =1.189, df=226, P =0.236) and slopes at (digit: r =0.041, df=226, P =0.541) or near the prediction (limb 95% confidence interval=−1.08 to −1.02) ( Fig. 3a–e ). 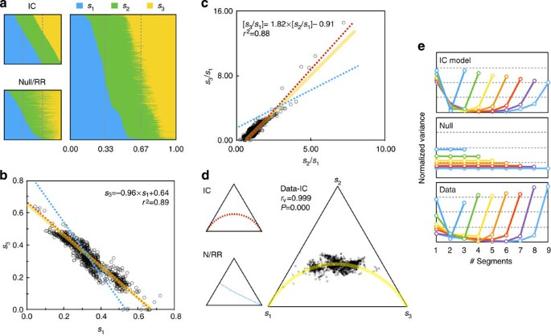Figure 3: Three-segment phalangeal and limb proportions exhibit patterning consistent with the IC model. (a) Proportional data distributions sorted in ascending order for the first segment (s1). Linear estimates (yellow line) for the PD tradeoff (b) and ratio prediction (c) compared with model (red) and null (AD, blue) predictions. (d) Ternary diagrams with estimated PC1 (IC=inhibitory cascade, red; N/RR=null/random relay, blue). Each point represents a single limb or phalangeal segment series or block. (e) Normalized variance profiles for segments from three to nine segments in null, observed data and IC model. Figure 3: Three-segment phalangeal and limb proportions exhibit patterning consistent with the IC model. ( a ) Proportional data distributions sorted in ascending order for the first segment ( s 1 ). Linear estimates (yellow line) for the PD tradeoff ( b ) and ratio prediction ( c ) compared with model (red) and null (AD, blue) predictions. ( d ) Ternary diagrams with estimated PC1 (IC=inhibitory cascade, red; N/RR=null/random relay, blue). Each point represents a single limb or phalangeal segment series or block. ( e ) Normalized variance profiles for segments from three to nine segments in null, observed data and IC model. Full size image To facilitate comparison among segmental types of varying lengths (for example, long digit and somite series), we next broke global series for the comparative data sets into all adjacent three-segment ‘local’ series and blocks (segment n =3–28, sample N =2,166) ( Supplementary Fig. 5a–f ). Again, we found that the middle segment or block averaged ~1/3 (s n +1 =0.343±0.014), variance was significantly lower compared with adjacent segments (Levene’s test, P <0.001) and there was an associated tradeoff between any first ( s n ) and third ( s n +2 ) segment proportion, regardless of position in the series ( s n +2 =−0.91· s n +0.63, r 2 =0.879, P <0.001). Moreover, the segment ratios were significantly correlated (that is, [ s n +2 ]/[ s n ]=1.75·[ s n +1 ]/[ s n ]−0.78, r 2 =0.826, P <0.001), indicating that the sizes of any first two segments were a highly significant predictor of the subsequent third segment size. When we evaluated the comparative data in a multivariate framework, we found that eigenvectors from the comparative data were significantly better correlated with the IC model predictions than with the alternative null models (PC1 angle=1.49, r v =0.9997, Fisher- z =4.36, P <0.001) ( Fig. 4 ; Supplementary Tables 3 ). 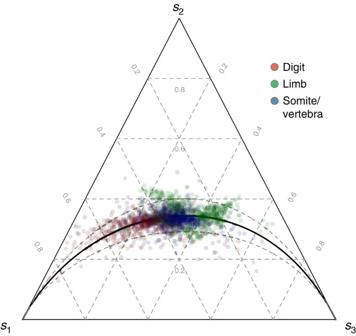Figure 4: Macroevolutionary diversity in phalanges, limb, somite and vertebral segment proportions exhibit similar properties. Ternary diagram showing comparative species-level variation in 2,000+ segment proportions in various structures reported in the text. Solid line shows the multivariate regression with 95% confidence interval denoted by the dashed lines. Figure 4: Macroevolutionary diversity in phalanges, limb, somite and vertebral segment proportions exhibit similar properties. Ternary diagram showing comparative species-level variation in 2,000+ segment proportions in various structures reported in the text. Solid line shows the multivariate regression with 95% confidence interval denoted by the dashed lines. Full size image Our results demonstrate that the IC provides a common explanatory framework for the generation of scale-free size variation (that is, proportions) in a variety of segmented structures in vertebrates. Previous work on this phenomenon was limited to teeth [14] , [24] , [25] , and it was unclear whether the activator interactions proposed in the IC also predicted ‘rules’ applicable to other sequentially forming structures. Given the explanatory power of IC predictions for the results presented here, this model may be generalizable to a range of other structures and phylogenetically distant taxa. Importantly, this mechanism also appears to impact both short-term responses of population-level variation and long-term patterns of macroevolutionary diversity to selection, and thus should help explain variational bias in a range of structural phenomena. The puzzle of this result is, given the potential ubiquity of a relatively simple and common regulatory ‘logic’ and the subsequent limits on variation it entails, how is evolutionary diversity generated? In part this question results from the disparity between perceived and measurable diversity, the latter of which is substantially smaller than the former. That said, while the IC biases variation in a predictable manner, there are number of ways in which these ‘rules’ may be combined with other developmental processes to produce more complex patterns. These include: (1) the iterative use of simple segmentation rules as ‘sub-routines’ within hierarchical modules (for example, phalangeal segmentation occurs within limbs; and such modularity is also consistent with evolution of the mammalian vertebral column [26] ), (2) the shaping of cell number or volume into alternative shapes and (3) the use of later developmental events like growth to ‘fine tune’ outcomes on a regional basis ( Supplementary Fig. 6a–d ). For example, while vertebrae vary in size across regions and frequently alternate in size, evidence from growth in a number of species suggests this results from later differential growth [27] , [28] , consistent with earlier constraints on somite-size patterning and proportions. We therefore hypothesize that an IC mechanism provides the initial pattern of proportional variation during segment formation, serving as a ‘foundation’ on which later variation may add or subtract [29] . That said, while later developmental processes such as differential growth may remodel proportions, the signal of the earlier segmentation event is not obliterated. We propose that activator/inhibitor ratios, broadly defined, are the mechanism for the evolutionary and developmental changes observed in segmented structures on both local and global (whole structure) scales. The shared developmental rules and quantitative predictions of the IC model suggest underlying commonalities that may help inform previous models of limb, digit and somite formation by recasting them in an activator–inhibitor framework. For example, more explicit reaction-diffusion models of proximo-distal axis formation [30] , [31] may be more accurate than classic descriptions such as the ‘progress zone’, ‘early specification’ or ‘two-signal’ models (discussed in ref. 15 ), which propose that individual segments initially form as a function of time balanced by inhibitory signals from the distal limb tip. Somitogenesis has likewise been conceived of proceeding via a ‘clock’ that interacts with an inhibitory ‘wavefront’ [16] , and newer studies suggest that the clock period changes with shortening of the unorganized (presomitic) mesoderm [32] and is partly self-organizing [33] . In both cases, the clock determining condensation formation can be conceived of as an auto-regulatory activator process that is balanced by an auto-regulatory inhibitory signal, each of which presumably can be varied. Supporting this idea, we note that up or downregulation of the inhibitory signal in somitogenesis [16] leads to localized changes in proportions of individual segments that we would predict are quantitatively consistent with the IC model. Our results contribute to increasing evidence that activator–inhibitor interactions are involved in limb, digit and somite segmentation, and could reflect a universal design principle [4] , [30] , [31] , [32] , [33] , [34] , [35] , but while confirmatory these results do not clarify the identity of the molecule(s) or the exact developmental mechanisms involved. We argue that the value of using the IC model is that, while previous models describe how segments form, they make no predictions about how they vary in size, and imply that elements are either independently formed or that segment proportions are largely the result of selection on later developmental events such as growth. Here we show that earlier events are crucial to the generation and patterning of evolutionary diversity. Moreover, commonalities in proportional outcomes indicate that knowledge of the specific molecules involved is likely less important than how they interact within a regulatory network. These results show how quantitative outcomes from comparative and experimental data are informative of the kinds of developmental interactions that are possible, and provide explicit predictions that will help inform future models of segment development and evolution. Specifically, the IC may provide a common framework, in a variety of developmental contexts, for predicting both short-term responses to selection in population-level variation and long-term evolvability and patterns of macroevolutionary diversity. Data To test our model against as many examples as possible, we collected segment size data from the limbs, phalanges, somites and vertebral columns of laboratory specimens, museum collections and previously published data sets for both limbs and digits. See Supplementary Data 1–11 for complete list of taxa, segment proportions and source information. Segment proportions were assessed using comparable proxies of size including: (i) length of the whole segments (for example, arm/leg, forearm/shank and manus/pes), (ii) maximum length of the skeletal elements (for example, ventral height of the vertebral body) or (iii) area/volume of segments. The exception to these was data from pigeons, in which the autopod measure did not include digit length, inflating stylopod and zeugopod estimates ( Supplementary Data 2 ). We note that although volume or cell number may be the most appropriate measure of size for the developmental phenomena we describe, variational properties and model predictions (for example, proximo-distal (PD) tradeoff) are not affected, regardless of the size measure used. Digit data was measured as the proportion of the proximal, middle and distal phalanx to total size of the phalangeal series, using both length measures and area of bone in dorsal/ventral view. For phalangeal chondrogenic condensation data, we collected normal chicken embryos at the end of digit segmentation (D11), stained for cartilage using Alcian blue and measured areas of segments in ImageJ. Alcian-stained chondrogenic condensations were measured as above and compared among treatment groups. We did not include the final phalanx (that is, ungual) in avians due to evidence that this segment represents a separate module in which a distal secondary ossification centre of dermal origin fuses to the final phalanx, complicating measures of initial size. This distal-most phalangeal segment, known as the ungual, may also be derived due to its association with secondary dermal ossification centres associated with claws and nails [36] , [37] . For total segment numbers of three or four, we utilized species-averaged data for each limb or digital ray. We used individual specimen data where total segments are >4. We considered forelimbs and hindlimbs in the same species to be independent data points, as well as each ray within a species autopod. For somite data, we collected avian embryos at HH8-10, and stained to improve visualization of the individual forming segments and measured two-dimensional area in ImageJ. Barrier experiment Tantalum foil implants were inserted into nascent pre-chondrogenic condensations of chick hindlimb digit IV on day 6–7. Embryos were collected at D10–11, fixed and Alcian stained as described above. Wound controls had foil barriers inserted and then removed about 1 min later. Area was measured as above ( Supplementary Data 1 ). Developmental model In a simplified IC model of activation and inhibition, the size of a segment is predicted by the equation: Where s is a segment (size or proportion), n is the number of the segment (from proximal to distal), a is the activator strength and i the inhibitor strength [14] . We assume a linear effect of activator to inhibitor. Solving this equation for a three-segment system yields segments sizes of: [ s 1 ]=1, and , and proportions are , and (ref. 14 ). Because , then and , and variance is predicted to be [ s 1 ]=[ s 3 ] and [ s 2 ]=0. This equation can be similarly solved for any n segments, and yields generalized predictions for segment proportion variation ( Supplementary Table 1 ; Supplementary Figs 1 and 2 ). For example, in the case of four segments: , , and . Notably, equation (1) generalizes for any three consecutive segments [ s n ]…[ s n+ 2 ], such that: In which case, total size of three consecutive segments is equivalent to: And thus the proportion of the middle segment [ s n +1 ] equals: It follows that the proportions of the remaining segments ( s n and s n+2 ) account for 2 / 3 of series size and function as a tradeoff. As an example, when a four-segment series (that is, [ s 1 – s 4 ]) is analysed as two local series (that is, [ s 1 – s 2 – s 3 ] and [ s 2 – s 3 – s 4 ]), each would be predicted to exhibit a middle segment proportion of 1 / 3 with reduced variance relative to a proximal-distal tradeoff. The global relationship would still be predicted to vary in a manner consistent with a four-segment series. This nested relationship between series of different lengths implies that segments interact locally with their direct neighbours, but because this effect is cumulative (that is, a ‘ratchet’) there is a global effect on the whole series ( Supplementary Fig. 5a ). Importantly, local and global effects enable the analysis of multi-segmented structures as series of ‘blocks’ of varying effective size. For global series of total segment number n , the average segment proportion equals 1/ n . If the first segment accounts for >2/ n of total proportional size, the ultimate segment is predicted to be negative, which implies a condensation cannot form. Furthermore, the first and ultimate segment proportions are predicted to tradeoff and exhibit equivalent variance. When plotted as a function of segment number, normalized segment variance is parabolic, with exponents following a power law relationship. In odd numbered segmental systems, the middle segment is predicted to be invariant and account for 1/ n of total proportions, where n is the total number of segments. For example, in a five-segment system ( n =5), [ s 3 ] is predicted to be ~ 1 / 5 , or ~14.3%, of total size ( Supplementary Fig. 2a,b ). Null models For the null models, we modelled three different assumptions about how segment sizes are generated and how proportions interact ( Supplementary Fig. 3a–o ).At first, we assumed that individual segment sizes are independently generated, thus we randomly generated vectors of length [1, n ] in which segment proportions were both unconstrained, uncorrelated, with a log normal distribution, where the mean and normalized variance of each segment is equivalent. Second, we utilized a ‘random relay’, in which we randomized the ratio of a and i between segments [14] ). In this case, covariance among segments still exists but is randomized in its direction, reflecting an inhibitory effect that is dependent on the segments involved rather than a constant function of the cascade. Third, we tested a simple ‘ascending–descending’ model in which segment proportions may be the same, increase or decrease, but do not alternate. We reasoned that this case described a general class of models in which segments interact in a constant direction (for example, same, up or down), but the magnitude of the effect varies between any given pair of segments. In this case, the IC model represents one specific set of possibilities in which the interaction effect between activation and inhibition is constant among all segments. Linear estimation We used reduced major axis to estimate linear parameters because all variables are measured with error. Test statistics for hypotheses of slope and elevation were based on modified ANCOVA for reduced major axis as estimated in the smatr3 package [38] ) in R [39] . We performed a centred log-ratio transformation on proportional series and report descriptive statistics (center and variance) for the compositional space [40] using both CoDaPack v.2.01.14 (ref. 41 ) and the R package compositions [42] . We calculated the variance for each segment series length ( n =3–7) for the comparative data, IC model and null predictions, and normalized for the total variance of the series. Principal components analysis We performed a robust principal components analysis (PCA) in a ternary compositional framework using the R package robCompositions [43] . A ‘robust’ PCA is similar to an ordinary PCA (that is, it is a method of ordination and data simplification), but differs in that it is less sensitive to outliers, thus increasing signal even in small sample sizes, which we justify due to the low dimensionality. We note that use of eigenvectors from a classical PCA would not alter the interpretation of results. ‘Ternary’ refers to the diagram utilized to represent the data type (that is, composed of three terms). The ‘compositional framework’ refers to the fact that proportional data considered as a whole (a ‘composition’) exhibit statistical properties that differs from classical measures due to the use of a shared denominator. The raw data undergo a centre-log-transform to place them in a new statistical ‘space’ before implementation of the robust PCA. We calculated the angle between the observed eigenvectors and those predicted by the IC model and the alternative null models, as well as the associated vector correlation ( r v ) and Fisher- z score (because correlations are not normally distributed). We tested the null hypothesis that the observed-IC correlation was not higher than the observed-null correlations by randomly generating null populations, calculating the associated eigenvector and then calculating the number of times the observed-null z -score exceeded that of the observed-IC using Monte Carlo simulation (10,000 bootstrap replicates) [44] implemented as a custom algorithm in R [39] . How to cite this article: Young, N. M. et al. Shared rules of development predict patterns of evolution in vertebrate segmentation. Nat. Commun. 6:6690 doi: 10.1038/ncomms7690 (2015).